A photon thermal diode A thermal diode is a two-terminal nonlinear device that rectifies energy carriers (for example, photons, phonons and electrons) in the thermal domain, the heat transfer analogue to the familiar electrical diode. Effective thermal rectifiers could have an impact on diverse applications ranging from heat engines to refrigeration, thermal regulation of buildings and thermal logic. However, experimental demonstrations have lagged far behind theoretical proposals. Here we present the first experimental results for a photon thermal diode. The device is based on asymmetric scattering of ballistic energy carriers by pyramidal reflectors. Recent theoretical work has predicted that this ballistic mechanism also requires a nonlinearity in order to yield asymmetric thermal transport, a requirement of all thermal diodes arising from the second Law of Thermodynamics, and realized here using an ‘inelastic thermal collimator’ element. Experiments confirm both effects: with pyramids and collimator the thermal rectification is 10.9±0.8%, while without the collimator no rectification is detectable (<0.3%). Energy is one of the dominant issues of modern times, and the large majority of it passes through the thermal domain [1] . Traditional thermal engineering is based on the paradigm of linear thermal elements, such as thermal resistors ( R ) and capacitors ( C ), and in this sense lags many decades behind electrical engineering, which has benefited greatly from ingenious applications of nonlinear elements. The most basic such element would be a thermal rectifier. Following one common convention [2] , [3] , we define the thermal rectification as where Q Fwd and Q Rev are the heat transfers under the same thermal bias Δ T = T H − T C but different directions: Forward (Fwd) and reverse (Rev). Regardless of the type of energy carrier, all thermal rectifiers require two key ingredients ( Fig. 1 ): asymmetry and nonlinearity [4] , [5] , [6] , [7] , [8] , [9] . Classical thermal diodes include natural convection in a gravitational field (molecular gases) and a Fourier Law mechanism exploiting temperature-dependent thermal conductivities (electrons and phonons) [7] , [10] . Additional thermal rectification mechanisms, including atomistically based proposals [4] , [5] , [6] , [11] , have been summarized in refs 7 , 12 . Within radiation heat transfer (photons), to our knowledge, rectification has not been experimentally established by any mechanism, classical or otherwise, although recent theoretical work has suggested far-field [12] and near-field [13] , [14] mechanisms exploiting temperature-dependent total emissivity, ε ( T ). 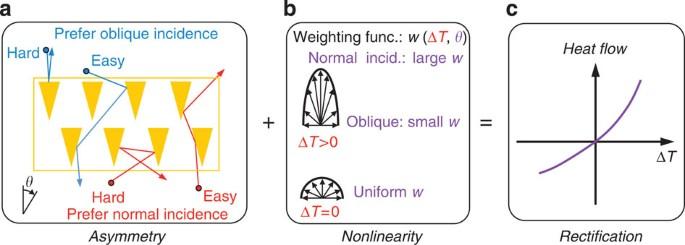Figure 1: The two key ingredients of a photon thermal diode: asymmetry and nonlinearity. (a) Asymmetry arises from angle-dependent transmission through the test section containing pyramidal reflectors: from bottom to top, transmission is higher for energy carriers with normal incidence, while from top to bottom, transmission is favoured for carriers of oblique incidence. (b) The nonlinearity arises because the emission from the hot reservoir (not shown) has an angular weighting that is also bias-dependent due to the ‘inelastic thermal collimator’. At zero thermal bias (ΔT=0), the angular weighting is nearly uniform (that is, Lambertian), while for non-zero thermal bias (ΔT>0), the emission becomes increasingly forward-peaked. (c) The combined effect is thermal rectification. See alsoSupplementary Notes 1–4. Figure 1: The two key ingredients of a photon thermal diode: asymmetry and nonlinearity. ( a ) Asymmetry arises from angle-dependent transmission through the test section containing pyramidal reflectors: from bottom to top, transmission is higher for energy carriers with normal incidence, while from top to bottom, transmission is favoured for carriers of oblique incidence. ( b ) The nonlinearity arises because the emission from the hot reservoir (not shown) has an angular weighting that is also bias-dependent due to the ‘inelastic thermal collimator’. At zero thermal bias (Δ T =0), the angular weighting is nearly uniform (that is, Lambertian), while for non-zero thermal bias (Δ T >0), the emission becomes increasingly forward-peaked. ( c ) The combined effect is thermal rectification. See also Supplementary Notes 1–4 . Full size image Here we present a new mechanism of photon thermal rectification, inspired by a pioneering ballistic electrical diode [15] and previous explorations of ballistic phonon thermal diode [8] , [9] , [16] , [17] , [18] . Figure 1 shows the basic concept, described in more detail in the Supplementary Notes 1–4 . Owing to the taper of the pyramidal mirrors, photons of near-normal incidence ( θ ≈0°) have higher transmission for trajectories from bottom to top than from top to bottom. However, the trend is opposite for trajectories entering the test section at highly oblique incidence ( θ approaching 90°). At equilibrium, these effects must exactly cancel, a fundamental requirement of the second Law of Thermodynamics (equivalently, conservation of optical etendue [19] ). As recently noted by ourselves [9] and others [8] , this further implies that the asymmetric structure of Fig. 1a alone [16] , [17] cannot show rectification even far away from equilibrium. A nonlinearity is also mandatory [4] , [5] , [6] , [7] , [8] , [9] , which we achieve through an ‘inelastic thermal collimator’ whose angle-dependent emission distorts as a function of the net thermal flux (see also Supplementary Notes 3 and 4 ). Here we experimentally demonstrate both the rectification effect and the necessity of the collimator. 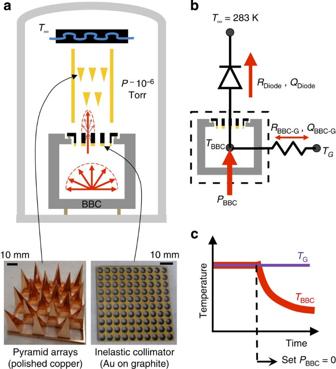Figure 2: Experimental concept. (a) A hot BBC (its guard heater and shields omitted for clarity) generates photons with a Lambertian distribution. The essential diode components are the inelastic thermal collimator and the test section with pyramidal mirrors. The depicted configuration is Fwd-biased, with Rev bias obtained by flipping the test section. (b) Energy balance applied to the BBC (dashed line): changes in stored thermal energy are balanced by the electrical heater (PBBC) and heat transfers through the diode (QDiode) and to/from the guard (QBBC-G). (c) Lumped cooling scheme: after stabilizing the BBC and guard atTBBC=TG=573 K, the BBC power is shut down, whileTGheld constant.QDiodeis extracted from the resulting BBC cooling curve. Experimental design Figure 2a shows the experimental concept. Photons are emitted from a graphite blackbody cavity (BBC) at T BBC =573 K, which offers a well-defined boundary condition with a nearly Lambertian emission (for design details see Supplementary Note 1 ). The cold side of the radiation field is maintained at T ∞ =283 K using a water-cooled black plate. For asymmetric scatterers we use highly polished copper pyramids, chosen for their high infrared reflectivity. As in Fig. 1a , photons incident towards the pyramids’ peaks have higher transmission for normal incidence, while photons incident towards their bases have higher transmission for oblique incidence (see Supplementary Figs 2 and 3 for further verification). Figure 2: Experimental concept. ( a ) A hot BBC (its guard heater and shields omitted for clarity) generates photons with a Lambertian distribution. The essential diode components are the inelastic thermal collimator and the test section with pyramidal mirrors. The depicted configuration is Fwd-biased, with Rev bias obtained by flipping the test section. ( b ) Energy balance applied to the BBC (dashed line): changes in stored thermal energy are balanced by the electrical heater ( P BBC ) and heat transfers through the diode ( Q Diode ) and to/from the guard ( Q BBC-G ). ( c ) Lumped cooling scheme: after stabilizing the BBC and guard at T BBC = T G =573 K, the BBC power is shut down, while T G held constant. Q Diode is extracted from the resulting BBC cooling curve. Full size image The second key ingredient is the nonlinearity, realized here through an ‘inelastic thermal collimator’ (see also Supplementary Notes 3 and 4 ). This differs quite fundamentally from a conventional optical collimator. The inelastic collimator must absorb a substantial portion of the incident photons and re-emit them at a lower energy, an inelastic interaction that provides bias-dependent angular weighting of emission as depicted in Figs 1b and 2a . In contrast, a conventional optical collimator ideally interacts with the photon field only by reflection and/or refraction, which as purely elastic processes are incapable of providing the needed nonlinearity [8] , [9] . To realize an inelastic thermal collimator in practice, we created a perforated graphite plate coated with gold film as an infrared reflector on the side facing the BBC ( Fig. 2a ). The collimator is mounted to the BBC using weak thermal links. These features ensure that, whenever the diode experiences substantial thermal bias, the temperature of the collimator floats to an intermediate value, which is significantly lower than that of the BBC (for example, T col ~473 K when T BBC =573 K and T ∞ =283 K). Then, owing to the open holes in the collimator, for angles close to θ ≈0° many of the photons entering the pyramid test section were emitted from the BBC core at T BBC . However, photons entering at oblique angles are much more likely to have been emitted from the internal cylindrical surfaces of the collimator holes, with lower intensity since T col < T BBC . The greater the thermal bias, the larger the difference between T col and T BBC , and thus the greater the angular distortion of the intensity incident on the pyramids. The configuration shown in Fig. 2a is Fwd-biased: when the BBC is hot, photons emitted normally have more intensity and are relatively easy to transmit through the pyramidal test section. Similarly, flipping the test section upside down creates Rev bias: the collimator emission is still weighted towards normal incidence; however, this is now relatively difficult to transmit through the test section. The result is thermal rectification. The experimental design ensures that convection and conduction losses from the BBC are below 0.1% (see Supplementary Note 1 ). To minimize radiation heat losses from the BBC exterior (<1%), we surround it with five concentric radiation shields and an active guard heater. A kinematic coupling between test section and BBC ensures positioning accuracy and repeatability when flipping the test section between polarities. The BBC and its guard each have two independent heater loops ( Supplementary Fig. 1b ), each typically stable to within ±0.5 K, with maximum differences of 1.5 K among these four heater zones as measured by six thermocouples. This experiment requires highly accurate measurements of the heat transfer through the test section, Q diode , under Fwd and Rev biases. Direct evaluation of the steady-state BBC power from the heaters’ current I and voltage V was found to be impractical because of the highly oscillatory nature of PWM-switched AC electricity. Instead we implemented the lumped cooling method [20] depicted in Fig. 2b,c . First, the BBC and guard are both stabilized at 573 K. Then for times t >0, the BBC heaters are turned off ( P BBC =0), while the guard is maintained at its original temperature. From the time-dependent cooling curve ( Fig. 2c ) we extract Q diode as follows. The excellent shielding between BBC and guard ensures Q BBC-G ≪ Q diode . This approaches the perfect-shield limit (see Supplementary Note 6 ), whereby the BBC energy balance of Fig. 2b simplifies to where C BBC is the thermal capacitance of the BBC (with SI units J K −1 ). In our experimental regime, the perfect-shield approximation of equation (2) agrees with exact numerical solutions to within 0.1% (see Supplementary Note 6 ), and also brings several experimental advantages. Most importantly, the cooling curve becomes independent of T G and R BBC-G ; therefore, the final results are insensitive to drifts or fluctuations in these quantities. In addition, Q diode comes directly from the cooling rate, |d T BBC /d t |, which is measured with much better accuracy than the electrical power P BBC =[ IV ] BBC . Furthermore, although quantifying Q diode requires an estimate for C BBC based on the BBC’s geometry and specific heat capacity [21] , C BBC is a common parameter for both Fwd and Rev biases, and thus cancels out in equation (1). Thus, rectification is calculated directly from the cooling curves using where both derivatives are evaluated numerically over the same temperature range. This differential expression is also advantageous because many possible errors are common-mode and thus would cancel out. Thermal transport results We performed two types of experiments to verify the key predictions [8] , [9] that both asymmetry and nonlinearity are required in a ballistic thermal rectifier. First, we performed six control experiments with the test section but without the collimator. These tests quantify the repeatability of the experiment and rule out potential artifacts, and check the theoretical prediction that asymmetry alone is insufficient for rectification. Between every trial, the test section is manually removed and replaced to capture effects of possible misalignment errors. The open points in Fig. 3a show two such control experiments, with the test section in Fwd and Rev biases. The BBC heater is turned off at 573 K, and we allow a 4-K buffer before defining t =0 to ensure the system has fully transitioned to its free-cooling trajectory. To better detect any differences between the curves, in Fig. 3b we plot the cooling rate, |d T BBC /d t |, evaluated numerically over a 10-point (10 min) moving average. Both panels confirm that these two control experiments are virtually indistinguishable from each other. To conveniently describe each trial with a single number, we average the cooling rate from 569 to 553 K and calculate the corresponding heat flow through the diode using equation (2). The results for three trials each of Fwd and Rev biases are plotted in Fig. 3c using the unfilled columns. Comparing the Fwd bias and Rev bias trials among themselves shows that the repeatability of these experiments is better than 0.8% (s.d.). Having quantified the noise floor of this apparatus, we next compare the average Q Diode,Fwd to the average Q Diode,Rev in these six control experiments. The difference of 0.3% is well within experimental uncertainty. Thus, as expected [8] , [9] , this is the first experimental confirmation that ballistic thermal rectification is not possible through asymmetric scattering alone. 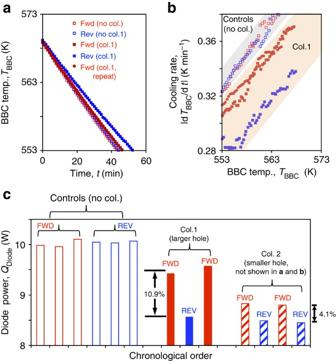Figure 3: Experimental results. (a) Cooling curves for representative experiments without (open points: controls) and with (filled points) the inelastic thermal collimator. (b) Cooling rates calculated fromausing a 10-point moving average. Symbols as ina. The two control experiments (shaded in grey) are virtually indistinguishable from each other, while the three experiments with the collimator (shaded in orange) are clearly separated. (c) Diode heat transfers calculated from equation (2) by averaging the cooling rate inbfrom 569 to 553 K, and including additional trials. These key results demonstrate how thermal rectification requires both asymmetry and nonlinearity. Another collimator (Col. 2: striped bars) with narrower holes shows similar results, but as expected degrades the rectification (Col. 2 data omitted froma,bfor clarity). Figure 3: Experimental results. ( a ) Cooling curves for representative experiments without (open points: controls) and with (filled points) the inelastic thermal collimator. ( b ) Cooling rates calculated from a using a 10-point moving average. Symbols as in a . The two control experiments (shaded in grey) are virtually indistinguishable from each other, while the three experiments with the collimator (shaded in orange) are clearly separated. ( c ) Diode heat transfers calculated from equation (2) by averaging the cooling rate in b from 569 to 553 K, and including additional trials. These key results demonstrate how thermal rectification requires both asymmetry and nonlinearity. Another collimator (Col. 2: striped bars) with narrower holes shows similar results, but as expected degrades the rectification (Col. 2 data omitted from a , b for clarity). Full size image Finally, we measure the complete device with pyramidal test section and inelastic thermal collimator. The collimator geometry was guided by a simple model (see Supplementary Note 5 ), with a pore aspect ratio H / D =1 and areal porosity chosen to be as large as practical (here 0.55). As summarized in Fig. 3a,b , with this collimator in place the measurements now show that the Fwd bias configuration (red filled squares) now clearly cools faster than the Rev bias case (blue filled squares). For example, at a BBC temperature of 563 K, Fig. 3b shows that the BBC cooled at 0.352 K min −1 in Fwd bias, but 0.314 K min −1 in Rev bias. Repeatability was confirmed after the Rev bias test by flipping the test section again and re-measuring Fwd bias, with very good consistency (red filled circles). Thus, as summarized in Fig. 3c using the filled columns, this ballistic thermal diode showed a rectification γ =10.9%, far above the uncertainty floor of 0.8%. To further verify the effect, the experiment was repeated using a second collimator with the same thickness and areal porosity but holes of half the diameter ( H / D =2). A simple model of the inelastic thermal collimator ( Supplementary Note 5 ) predicts that this should degrade the overall rectification performance. This was confirmed by experiment: the striped columns in Fig. 3c show that the resulting heat transfer was again asymmetric and highly repeatable among four trials, and as expected the rectification was significantly reduced ( γ =4.1%). Lastly, Fig. 1b and Supplementary Fig. 4 qualitatively suggest that the distorting effect of the inelastic thermal collimator is degraded at lower thermal bias. This trend is also seen in the simple collimator model ( Supplementary Fig. 8 ) and confirmed by the experiment. As shown in Fig. 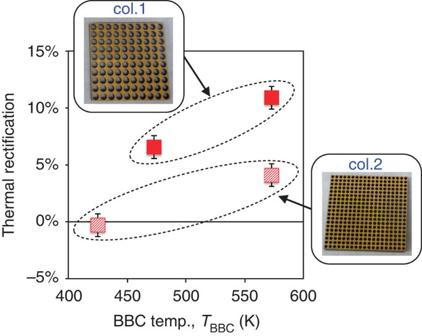Figure 4: Bias-dependent thermal rectification. These experimental results confirm the trends presented inSupplementary Fig. 4: rectification increases with thermal bias.T∞=283 K for all measurements. 4 , for Collimator 1 the rectification decreases from 10.9% at T BBC =573 K to 6.6% at T BBC =473 K, while keeping T ∞ fixed at 283 K. Similar trends are observed for Collimator 2, with rectification decreasing from 4.1% at 573 K to below the noise threshold at 425 K. Figure 4: Bias-dependent thermal rectification. These experimental results confirm the trends presented in Supplementary Fig. 4 : rectification increases with thermal bias. T ∞ =283 K for all measurements. Full size image The results in Fig. 3 represent the first experimental demonstration of a photon thermal diode using any mechanism. This is also the first demonstration of the two-terminal ballistic thermal rectification mechanism [8] , [9] , [16] , [17] for any carrier type, and in principle is generalizable to other ballistic carriers including electrons and phonons, for example, using pyramidal quantum dots [22] , sawtooth nanowires [16] , [17] , [23] or microfabricated structures (see Supplementary Note 7 ). Highly effective thermal rectifiers could find numerous applications in thermal engineering. Many arise from electrical analogues [24] . For example, in solar-thermal power, a temperature doubler (analogous to a voltage doubler) can exploit nighttime cold temperatures as well as daytime highs to increase the average temperature difference driving a heat engine, increasing both efficiency and power output [9] , [25] . A thermal diode’s clamping functionality could be useful for thermal regulation of building envelopes [26] , as well as thermal protection of delicate components in electrical hardware, spacecraft thermal shielding and satellite radiators. Thermal diodes are also a fundamental element for logic operations; besides the suggestion of thermal information processing [27] this can also benefit power generation, since a suitable array of thermal diodes can automatically pick out only the hottest of sources and coldest of sinks. How to cite this article: Chen, Z. et al . A photon thermal diode. Nat. Commun. 5:5446 doi: 10.1038/ncomms6446 (2014).